The stem cell factor/Kit signalling pathway regulates mitochondrial function and energy expenditure Cell growth is tightly coupled with mitochondrial biogenesis in order to maintain energy and organelle homeostasis. Receptor tyrosine kinase Kit and its ligand, stem cell factor (SCF), play a critical role in the growth and survival of multiple cell lineages. Here we report that the expression of SCF and Kit in adipose tissues is responsive to food availability and environmental temperature, and is altered in obese mice and human patients. Mice carrying a loss-of-function mutation in Kit develop obesity as a result of decreased energy expenditure. These phenotypes are associated with reduced PGC-1α expression and mitochondrial dysfunction in brown adipose tissue and skeletal muscle. We further demonstrate that SCF/Kit directly promotes Ppargc1a transcription and mitochondrial biogenesis. Blocking Kit signalling in mice decreases PGC-1α expression and thermogenesis, while overexpressing SCF systemically or specifically in brown adipose tissue increases thermogenesis and reduces weight gain. Collectively, these data provide mechanistic insight into the regulation of mitochondrial function by SCF/Kit signalling and lay a foundation for exploring SCF/Kit signalling as a therapeutic target for metabolic diseases. Energy expenditure mainly takes the forms of basal metabolism, adaptive thermogenesis and physical activity [1] . Obesity develops when energy intake exceeds total body energy expenditure [2] . Targeting energy expenditure is emerging as an alternative approach to control obesity in addition to decreasing energy intake. Cellular energy expenditure takes place largely within the mitochondria, where fuels are oxidized and energy is either stored as ATP or released as heat [1] . There are multiple mechanisms underlying heat production by uncoupled mitochondrial respiration, one of which is mediated by uncoupling proteins (UCPs). Specifically expressed in brown and beige/bright adipocytes, UCP1 is required to mediate adaptive thermogenesis [3] , [4] , [5] . Nevertheless, UCP1-independent processes exist to regulate energy expenditure [6] , [7] , [8] . Increasing evidence indicates that mitochondrial dysfunction is closely associated with metabolic disorders, such as obesity, insulin resistance and ageing [9] , [10] . Peroxisome proliferator-activated receptor-γ (PPARγ) coactivator-1α (PGC-1α, encoded by the Ppargc1a gene) has emerged as the master regulator of mitochondrial biogenesis and function [11] . PGC-1α activates mitochondrial biogenesis through stimulating mitochondrial transcription factor A (TFAM) and nuclear respiratory factors (NRFs), key regulators of mitochondrial DNA (mtDNA) replication/transcription [12] . PGC-1α co-activates PPARγ and thyroid hormone receptor (TR) on Ucp1 promoters to stimulate adaptive thermogenesis [13] . PGC-1α also triggers mitochondrial biogenesis in skeletal and cardiac muscle [14] , [15] . Consistent with these findings, PGC-1α deficiency leads to multi-organ metabolic defects, including obesity, cold intolerance, hepatic steatosis, glucose imbalance and muscle dysfunction [16] , [17] . Cellular growth controlled by cytokines and growth factors requires coordinated modulation of bioenergetics and mitochondrial function. Therefore, it is not surprising that mitochondrial function is tightly controlled by cytokines/growth factors to meet diverse energy demands [18] , [19] , [20] , [21] . Nevertheless, mechanistic studies are required to understand how cytokines/growth factors integrate the regulation of mitochondrial and cellular functions, and to determine their physiological and pathological significance at the whole-organism level. Signalling of stem cell factor (SCF, also known as Kit ligand, encoded by the Kitl gene) and its receptor Kit (encoded by the Kit gene) is critical for multiple lineages of stem/progenitor cells [22] . Loss-of-function mutations of either gene cause deficiencies/defects in melanocytes, mast cells, germ cells and hematopoietic cells [23] , while gain-of-function mutations are known to be causes of mastocytosis, gastrointestinal stromal tumours, germ-cell tumours and leukaemia [22] . Recently, SCF has been shown to generate brown adipocytes from human pluripotent stem cells, in collaboration with several other hematopoietins [24] . Here we report that SCF/Kit regulates mitochondrial function and energy homeostasis by modulating PGC-1α expression. Kit mutant mice develop obesity as a result of decreased mitochondrial biogenesis and energy expenditure. Our findings identify SCF/Kit signalling as a novel pathway regulating mitochondrial function and energy expenditure, shedding light on new strategies for the treatment of obesity and related diseases. SCF/Kit expression is altered in obese animals and humans We first examined the transcription of Kitl and Kit in key metabolic tissues in high-fat-diet (HFD)-induced obese mice. Though not changed in the arcuate nucleus of the hypothalamus, liver, muscle or gonadal white adipose tissue (WAT), mRNA level of Kitl is increased in the brown adipose tissue (BAT) in HFD mice ( Fig. 1a ). While Kit expression is significantly downregulated in both BAT and WAT in HFD mice, no difference in Kit transcription is observed in other tissues examined ( Fig. 1b ). 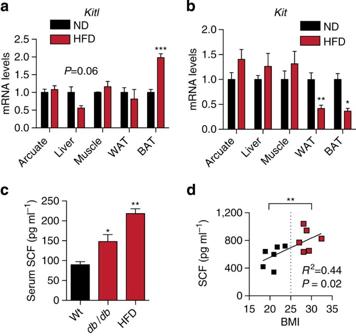Figure 1: Expression ofKitlandKit. (a)Kitland (b)KitmRNA levels in tissues from 6-month-old normal diet- (ND) and HFD-fed mice (n=5). (c) Serum levels of SCF in age-matched male wild-type,db/dband HFD mice (n=4). (d) Serum levels of SCF in humans. Data are shown as mean±s.e.m. *P<0.05; **P<0.01; ***P<0.001 by two-tailed Student’st-test (a,b,d) or one-way ANOVA followed with a Bonferroni’spost hoctest (c). Figure 1: Expression of Kitl and Kit . ( a ) Kitl and ( b ) Kit mRNA levels in tissues from 6-month-old normal diet- (ND) and HFD-fed mice ( n =5). ( c ) Serum levels of SCF in age-matched male wild-type, db / db and HFD mice ( n =4). ( d ) Serum levels of SCF in humans. Data are shown as mean±s.e.m. * P <0.05; ** P <0.01; *** P <0.001 by two-tailed Student’s t -test ( a , b , d ) or one-way ANOVA followed with a Bonferroni’s post hoc test ( c ). Full size image Consistent with these observations, serum levels of SCF are elevated in both HFD mice and obese/diabetic db / db mice ( Fig. 1c ). We also measured serum SCF in a cohort of human patients. SCF levels are positively correlated with body mass index (BMI), and are significantly elevated in the overweight group (BMI>25) compared with the lean group (BMI<25) ( Fig. 1d ). These data suggest that the SCF/Kit pathway is dysregulated upon metabolic overload. Increased adiposity in Kit mutant mice To determine the physiological role of Kit, we analysed the metabolic phenotypes of the Wps mouse strain, which carries a loss-of-function mutation in the Kit gene [25] . The Wps mutation does not affect the splicing of GNNK− versus GNNK+ Kit , but does significantly inhibit tyrosine kinase activity and downstream Akt and Erk signalling of Kit both in vitro and in vivo ( Supplementary Fig. 1 ) [26] . Both male and female homozygous Wps/Wps mice show increased body weight starting at the age of 3 and 4 months, respectively ( Fig. 2a,b ). Male heterozygous Wps /+ mice also have slightly increased body mass. To determine the source of the weight gain, we measured the body composition of 10-month-old mice. Fat weight and fat percentage are elevated in Wps / Wps mice, while the lean mass remains unchanged compared with wild-type mice ( Fig. 2c,d ). Consistent with increased adiposity, the mutant mice have higher levels of triglyceride (TG) and free fatty acids (FFAs) in the serum ( Fig. 2e,f ). We then assessed glycemic control in the mutant mice. Compared with wild-type controls, Wps/Wps mice exhibit glucose intolerance and insulin insensitivity, although the basal- and fasting glucose levels are normal ( Fig. 2g,h ). Fasting- and glucose induced-insulin levels are comparable between wild-type and Wps/Wps mice ( Fig. 2i ), suggesting that the Wps / Wps mice have peripheral insulin resistance. 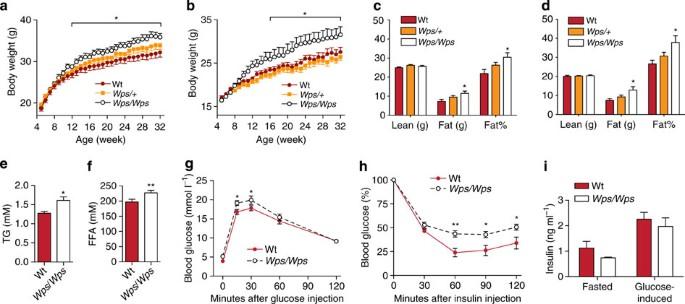Figure 2: Increase adiposity and impaired glucose homeostasis inWpsmice. (a,b) Growth curves of (a) male and (b) female wild-type andWpsmice (n=7–11). (c,d) Body compositions of 10-month-old (c) male and (d) female wild-type andWpsmice are shown (n=7–11). (e,f) Blood serum levels of (e) TG and (f) FFAs from overnight-fasted male mice (n=7–8). (g) Glucose tolerance test (GTT) of 6-month-old male mice (n=7–8). (h) Insulin tolerance test (ITT) of 6-month-old male mice (n=7–8). (i) Blood insulin levels of overnight-fasted and glucose-injected (i.p.) mice (n=3). Data are shown as mean±s.e.m. *P<0.05; **P<0.01 by two-tailed Student’st-test (a,b,e–h) or one-way ANOVA followed with a Bonferroni’spost hoctest (c,d). Figure 2: Increase adiposity and impaired glucose homeostasis in Wps mice. ( a , b ) Growth curves of ( a ) male and ( b ) female wild-type and Wps mice ( n =7–11). ( c , d ) Body compositions of 10-month-old ( c ) male and ( d ) female wild-type and Wps mice are shown ( n =7–11). ( e , f ) Blood serum levels of ( e ) TG and ( f ) FFAs from overnight-fasted male mice ( n =7–8). ( g ) Glucose tolerance test (GTT) of 6-month-old male mice ( n =7–8). ( h ) Insulin tolerance test (ITT) of 6-month-old male mice ( n =7–8). ( i ) Blood insulin levels of overnight-fasted and glucose-injected (i.p.) mice ( n =3). Data are shown as mean±s.e.m. * P <0.05; ** P <0.01 by two-tailed Student’s t -test ( a , b , e – h ) or one-way ANOVA followed with a Bonferroni’s post hoc test ( c , d ). Full size image We observed similar increases in body weight, fat percentage, adipocyte size and serum leptin level in another Kit mutant line, Wads [23] , suggesting that obesity is the general outcome in mice with loss-of-function Kit mutations ( Supplementary Fig. 2 ). Decreased energy expenditure in Kit mutant mice Obesity only develops when energy intake exceeds energy expenditure. Measurement of food intake in mice at young and old ages shows no difference between wild-type and Wps / Wps mice ( Fig. 3a ). Wps / Wps mice lose less body mass after food deprivation for 24 and 48 h ( Fig. 3b ), indicating lower energy expenditure in these mice. To test energy expenditure directly, gas exchange and activity levels in mice were monitored using metabolic cages ( Fig. 3c–e ). No difference in respiratory exchange ratio (RER) is observed, suggesting that similar amounts of carbohydrates and fat are consumed in wild-type and Wps / Wps mice ( Fig. 3c ). Heat production, on the other hand, is significantly decreased in Wps / Wps mice ( Fig. 3d ), which may contribute to the obesity in Wps / Wps mice. Wps / Wps mice also show decreased locomotor activity ( Fig. 3e ). 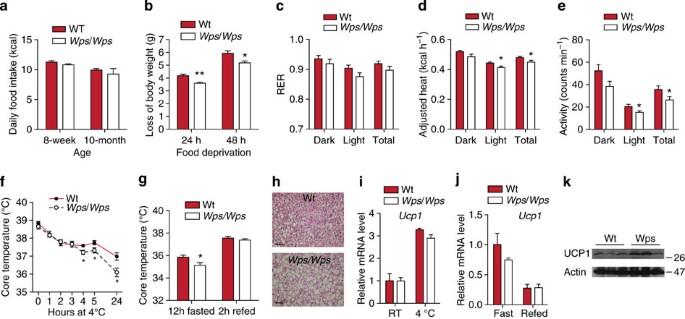Figure 3: Decreased energy expenditure inWps/Wpsmice. (a) Food intake of 8-week- and 10-month-old male mice (n=6). (b) Body-weight loss of 6-month-old male mice after 24 and 48 h of food deprivation (n=7). (c) RER, (d) ANCOVA analysis of body weight-adjusted heat production and (e) locomotor activity determined by metabolic cage study (n=17–18). (f) Rectal temperature of 6-month-old male mice after cold (4 °C) inducement (n=6–9). (g) Rectal temperature of 6-month-old male mice after 12 h fasting and 2 h refeeding (n=10–11). (h) Representative histology of BAT in wild-type andWps/Wpsmice. Scale bar, 50 μm. (i,j)Ucp1gene expression of (i) cold- and (j) fasting-treated mice (n=4). (k) UCP1 protein expression in BAT fromad libitumfed mice housed at room temperature. Data are shown as mean±s.e.m. *P<0.05; **P<0.01 by two-tailed Student’st-test. Figure 3: Decreased energy expenditure in Wps / Wps mice. ( a ) Food intake of 8-week- and 10-month-old male mice ( n =6). ( b ) Body-weight loss of 6-month-old male mice after 24 and 48 h of food deprivation ( n =7). ( c ) RER, ( d ) ANCOVA analysis of body weight-adjusted heat production and ( e ) locomotor activity determined by metabolic cage study ( n =17–18). ( f ) Rectal temperature of 6-month-old male mice after cold (4 °C) inducement ( n =6–9). ( g ) Rectal temperature of 6-month-old male mice after 12 h fasting and 2 h refeeding ( n =10–11). ( h ) Representative histology of BAT in wild-type and Wps / Wps mice. Scale bar, 50 μm. ( i , j ) Ucp1 gene expression of ( i ) cold- and ( j ) fasting-treated mice ( n =4). ( k ) UCP1 protein expression in BAT from ad libitum fed mice housed at room temperature. Data are shown as mean±s.e.m. * P <0.05; ** P <0.01 by two-tailed Student’s t -test. Full size image Wps / Wps mice have normal body temperature at basal conditions; however, their body temperature drops significantly lower than that of wild-type mice after cold exposure and fasting ( Fig. 3f,g ), suggesting a defect in thermogenesis in Wps / Wps mice. Histological analysis revealed an increase in number and size of lipid droplets in BAT of Wps / Wps mice ( Fig. 3h ). However, there is no change in Ucp1 transcript levels at all the conditions examined ( Fig. 3i,j ). In contrast, UCP1 protein levels increase slightly in Wps / Wps mice ( Fig. 3k ). We then housed the mice at thermoneutrality, when thermal stress is absent [27] , and measured energy expenditure ( Fig. 4a–c ). Wps / Wps mice generate much less heat than control mice during both light and dark phases ( Fig. 4a ). The decrease in heat production at thermoneutrality is larger than that at room temperature ( Fig. 3d ). RER or locomotor activity is not statistically different between the two genotypes ( Fig. 4b,c ). 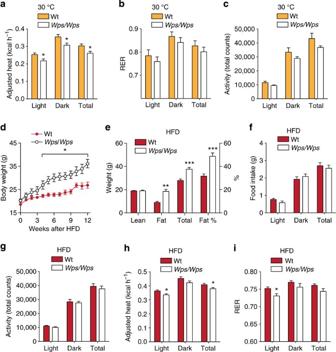Figure 4: Thermogenesis ofWps/Wpsmice at thermoneutrality and after HFD feeding. (a–c) Six-week-old Wt andWps/Wpsmice were housed at 30 °C for 1 week, and then were subjected for metabolic cage study at 30 °C for another 10 days. Data from the last 5 days were analysed and plotted (n=7–8). (a) Heat production adjusted to body weight using ANCOVA analysis, (b) RER and (c) locomotor activity. (d) Growth curve of 2-month-old mice after HFD feeding. (e) Body weight, lean mass, fat mass and fat percentage of mice after 12 weeks of HFD feeding (n=7). (f) Food intake, (g) locomotor activity, (h) heat production and (i) RER of HFD mice determined by metabolic cage study at room temperature (n=6–8). Data are shown as mean±s.e.m. *P<0.05 by two-tailed Student’st-test. Figure 4: Thermogenesis of Wps / Wps mice at thermoneutrality and after HFD feeding. ( a – c ) Six-week-old Wt and Wps / Wps mice were housed at 30 °C for 1 week, and then were subjected for metabolic cage study at 30 °C for another 10 days. Data from the last 5 days were analysed and plotted ( n =7–8). ( a ) Heat production adjusted to body weight using ANCOVA analysis, ( b ) RER and ( c ) locomotor activity. ( d ) Growth curve of 2-month-old mice after HFD feeding. ( e ) Body weight, lean mass, fat mass and fat percentage of mice after 12 weeks of HFD feeding ( n =7). ( f ) Food intake, ( g ) locomotor activity, ( h ) heat production and ( i ) RER of HFD mice determined by metabolic cage study at room temperature ( n =6–8). Data are shown as mean±s.e.m. * P <0.05 by two-tailed Student’s t -test. Full size image HFD feeding, which normally maximizes thermogenic capacity, further increases the gain of body weight and fat mass in Wps / Wps mice ( Fig. 4d,e ). Indirect calorimetric analyses demonstrate food intake and locomotor activity are similar between wild-type and mutant mice ( Fig. 4f,g ). However, energy expenditure in HFD Wps / Wps mice is downregulated, accompanied with a slight decrease in RER ( Fig. 4h,i ). Taken together, these data demonstrate that Wps mutation impairs the thermogenic capacity of BAT. Kit regulates mitochondrial function in adipose tissues Mitochondria are the powerhouse of the cell and are responsible for heat production. To evaluate mitochondrial function, we first examined the mitochondrial morphology of BAT using transmission electron microscopy (TEM) ( Fig. 5a ). Quantification of the mitochondria shows normal size, but decreased number and total area in Wps / Wps BAT ( Fig. 5b ). The defect in mitochondria precedes the onset of obesity ( Supplementary Fig. 3 ). There is also a reduction in mtDNA copy number in Wps / Wps BAT at the age of 12 weeks when no change in body weight is observed ( Fig. 5c ). Furthermore, there is a reduction in mitochondrial oxygen respiration when ATPase is inhibited by oligomycin in Wps / Wps mice, indicating a defect in the uncoupling function of Wps / Wps brown adipocytes ( Fig. 5d ). 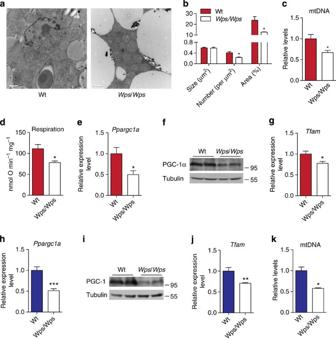Figure 5:Wpsmutation causes mitochondrial dysfunction in adipose tissues. (a) Representative TEM images of BAT from 5-month-old mice. Scale bar, 1 μm. (b) Size, number and total area of BAT mitochondria (n=3–4). (c) Relative mtDNA copy number in BAT from weight-matched 10–12-week-old mice (n=4). (d) Mitochondrial respiration rate in BAT from weight-matched 10–12-week-old mice (n=4). (e) Real-time quantification ofPpargc1amRNA levels in BAT (n=4). (f) Immunobloting of PGC-1α protein of BAT lysate from 6-week-old mice. (g) RelativeTfammRNA levels in BAT (n=4). (h) Relative mRNA and (i) protein levels of PGC-1α in WAT (n=4–5). (j) Relative expression ofTfammRNA level in WAT (n=4–5). (k) mtDNA copy number in WAT from weight-matched mice (n=7). Data are shown as mean±s.e.m. *P<0.05; **P<0.01 by two-tailed Student’st-test. Figure 5: Wps mutation causes mitochondrial dysfunction in adipose tissues. ( a ) Representative TEM images of BAT from 5-month-old mice. Scale bar, 1 μm. ( b ) Size, number and total area of BAT mitochondria ( n =3–4). ( c ) Relative mtDNA copy number in BAT from weight-matched 10–12-week-old mice ( n =4). ( d ) Mitochondrial respiration rate in BAT from weight-matched 10–12-week-old mice ( n =4). ( e ) Real-time quantification of Ppargc1a mRNA levels in BAT ( n =4). ( f ) Immunobloting of PGC-1α protein of BAT lysate from 6-week-old mice. ( g ) Relative Tfam mRNA levels in BAT ( n =4). ( h ) Relative mRNA and ( i ) protein levels of PGC-1α in WAT ( n =4–5). ( j ) Relative expression of Tfam mRNA level in WAT ( n =4–5). ( k ) mtDNA copy number in WAT from weight-matched mice ( n =7). Data are shown as mean±s.e.m. * P <0.05; ** P <0.01 by two-tailed Student’s t -test. Full size image PGC-1α is a master transcription cofactor regulating mitochondrial biogenesis and function that is itself regulated by transcription and extensive posttranslational modifications [11] , [28] . Consistent with the dysfunction of the mitochondria, both mRNA and protein levels of PGC-1α are reduced in Wps / Wps BAT before the appearance of the obese phenotype ( Fig. 5e,f ). The expression of PGC-1α target gene Tfam , a key regulator of mtDNA is also downregulated accordingly ( Fig. 5g ). Moreover, we observed the downregulation of mRNA and protein levels of PGC-1α in gonadal WAT of Wps / Wps mice ( Fig. 5h,i ). Tfam expression and mtDNA content are also decreased ( Fig. 5j,k ). Collectively, these data demonstrate that PGC-1α is downregulated and mitochondria are dysfunctional in Wps / Wps BAT and WAT. Wps Kit impairs mitochondrial function in skeletal muscle Skeletal muscle is another important tissue responsible for energy expenditure, mediating both physical activity and thermogenesis [1] . Decreased locomotor activity in Wps / Wps mice led us to examine mitochondrial function and PGC-1α expression in the muscle. Mitochondrial size, number, and total mass are all decreased in Wps / Wps soleus muscle as assessed by TEM ( Fig. 6a,b and Supplementary Fig. 3 ). mtDNA copy number drops nearly 50% in the soleus muscle of Wps / Wps mice compared with that of weight-matched wild-type mice at the age of 12 weeks ( Fig. 6c ). Measurement of the oxygen respiration of isolated mitochondria from soleus muscle demonstrated that State III oxygen consumption is impaired in Wps / Wps mice ( Fig. 6d ). 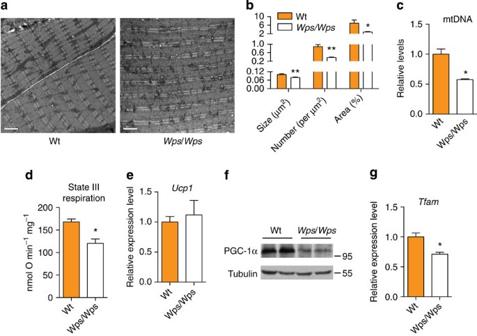Figure 6:Wpsmutation causes mitochondrial dysfunction in soleus muscle. (a) Representative TEM image of soleus muscle from 5-month-old mice. Scale bar, 2 μm. (b) Size, number and total area of mitochondria in soleus muscle (n=3–4). (c) mtDNA copy number in soleus muscle of weight-matched 10–12 week-old mice (n=4). (d) ADP-stimulated state 3 respiration of isolated soleus mitochondria from weight-matched 10–12 week-old mice (n=3). (e) Real-time quantification ofUcp1mRNA levels in soleus muscle (n=4–5). (f) Immunoblotting of PGC-1α in soleus muscle of 6 week-old mice. (g) RelativeTfammRNA levels in soleus muscle (n=4–5). Data are shown as mean±s.e.m. *P<0.05; **P<0.01 by two-tailed Student’st-test. Figure 6: Wps mutation causes mitochondrial dysfunction in soleus muscle. ( a ) Representative TEM image of soleus muscle from 5-month-old mice. Scale bar, 2 μm. ( b ) Size, number and total area of mitochondria in soleus muscle ( n =3–4). ( c ) mtDNA copy number in soleus muscle of weight-matched 10–12 week-old mice ( n =4). ( d ) ADP-stimulated state 3 respiration of isolated soleus mitochondria from weight-matched 10–12 week-old mice ( n =3). ( e ) Real-time quantification of Ucp1 mRNA levels in soleus muscle ( n =4–5). ( f ) Immunoblotting of PGC-1α in soleus muscle of 6 week-old mice. ( g ) Relative Tfam mRNA levels in soleus muscle ( n =4–5). Data are shown as mean±s.e.m. * P <0.05; ** P <0.01 by two-tailed Student’s t -test. Full size image No difference in Ucp1 mRNA is observed in soleus muscle ( Fig. 6e ). As found in adipose tissues, the expression of PGC-1α ( Fig. 6f ) and its target Tfam ( Fig. 6g ) in soleus muscle is significantly reduced in Wps / Wps mice. Taken together, we observed decreased PGC-1α expression and mitochondrial dysfunction in soleus muscle of Wps / Wps mice. SCF/Kit signalling regulates Ppargc1a transcription To directly test the regulation of Ppargc1a expression by Kit, we performed luciferase reporter assays in 3T3-L1 cells. Kit overexpression enhances the Ppargc1a promoter activity while the Wps mutant loses this effect ( Fig. 7a ). Meanwhile, SCF treatment induces the expression of endogenous Ppargc1a and Tfam in 3T3-L1 cells ( Fig. 7b,c ). The PI3K-Akt-mTOR and Ras-Erk pathways are the primary downstream targets of SCF/Kit signalling [22] . To determine which pathway(s) are important for the effect of SCF, 3T3-L1 cells were pretreated with inhibitors of PI3K, mTOR and MEK. Inhibition of PI3K (Wortmannin), mTOR (Rapamycin) or MEK (U0126) blocks the induction of Ppargc1a and Tfam transcription by SCF ( Fig. 7d,e ). A more selective PI3K inhibitor, ZSTK474 also prevents the effect of SCF on Ppargc1a and Tfam transcription in differentiated pre-brown adipocytes expressing wild-type Kit ( Fig. 7f,g ). However, brown adipocytes expressing Wps Kit are not responsive to SCF or ZSTK474 treatment ( Fig. 7f,g ), suggesting that the defect in SCF-induced PI3K signalling leads to Ppargc1a downregulation in Wps / Wps mice. Consistent with these observations, activation of Akt and Erk pathways by SCF is inhibited in BAT and soleus muscle from Wps/Wps mice ( Fig. 7h ). 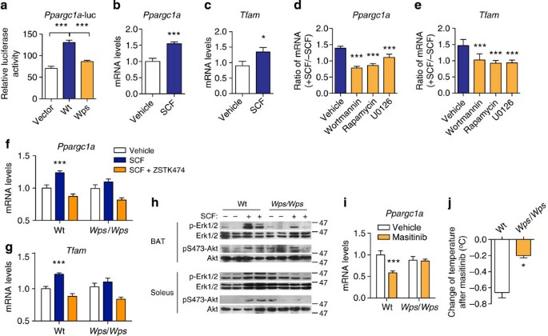Figure 7: SCF/Kit signalling regulatesPpargc1atranscription. (a)Ppargc1apromoter activity assay in the presence of Wt orWpsKit in 3T3-L1 cells (n=4). (b)Ppargc1amRNA levels after 6-h treatment of vehicle or SCF (n=3). (c)TfammRNA levels after treatment of vehicle or SCF (n=3). (d,e) 3T3-L1 cells were pretreated with inhibitors for PI3K (Wortmannin), mTOR (Rapamycin) or MEK (PD98059) followed by SCF treatment. The changes in the expression ofPpargc1a(d) andTfam(e) stimulated by SCF are shown (n=3). (f,g) Immortalized pre-brown adipocytes overexpressing wild-type orWpsKit were differentiated and treat with SCF in the absence or presence of ZSTK474, a selective PI3K inhibitor. Levels ofPpargc1a(f) andTfam(g) transcripts are shown. (h) Immunoblotting of proteins from BAT and Soleus muscle showing decreased Akt and Erk1/2 activation after SCF injection inWps/Wpsmice. (i) Pre-brown adipocytes from wild-type orWps/Wpsmice were treated with Masitinib, andPpargc1aexpression was determined. (j) C57Bl/6 mice (7–8-week-old) were i.p. injected with 50 mg per kg per day Masitinib for 3 days, and the changes in core body temperature was determined (n=4). Data are shown as mean±s.e.m. *P<0.05; ***P<0.001 by two-tailed Student’st-test (b,c,i,j) or one-way ANOVA followed with a Bonferroni’spost hoctest (a,d–g). Figure 7: SCF/Kit signalling regulates Ppargc1a transcription. ( a ) Ppargc1a promoter activity assay in the presence of Wt or Wps Kit in 3T3-L1 cells ( n =4). ( b ) Ppargc1a mRNA levels after 6-h treatment of vehicle or SCF ( n =3). ( c ) Tfam mRNA levels after treatment of vehicle or SCF ( n =3). ( d , e ) 3T3-L1 cells were pretreated with inhibitors for PI3K (Wortmannin), mTOR (Rapamycin) or MEK (PD98059) followed by SCF treatment. The changes in the expression of Ppargc1a ( d ) and Tfam ( e ) stimulated by SCF are shown ( n =3). ( f , g ) Immortalized pre-brown adipocytes overexpressing wild-type or Wps Kit were differentiated and treat with SCF in the absence or presence of ZSTK474, a selective PI3K inhibitor. Levels of Ppargc1a ( f ) and Tfam ( g ) transcripts are shown. ( h ) Immunoblotting of proteins from BAT and Soleus muscle showing decreased Akt and Erk1/2 activation after SCF injection in Wps / Wps mice. ( i ) Pre-brown adipocytes from wild-type or Wps / Wps mice were treated with Masitinib, and Ppargc1a expression was determined. ( j ) C57Bl/6 mice (7–8-week-old) were i.p. injected with 50 mg per kg per day Masitinib for 3 days, and the changes in core body temperature was determined ( n =4). Data are shown as mean±s.e.m. * P <0.05; *** P <0.001 by two-tailed Student’s t -test ( b , c , i , j ) or one-way ANOVA followed with a Bonferroni’s post hoc test ( a , d – g ). Full size image To test whether Kit kinase activity is necessary for the regulation of mitochondrial function, we treated pre-brown adipocytes with the Kit inhibitor, Masitinib. Masitinib selectively inhibits the level of Ppargc1a transcript in wild-type but not Wps / Wps adipocytes ( Fig. 7i ). More importantly, treatment of mice with Masitinib in vivo significantly reduces core body temperature of wild-type mice, but has minimal effect on Wps/Wps mice ( Fig. 7j ). Collectively, these data demonstrate that SCF/Kit signalling, through Akt and Erk pathways, regulates Ppargc1a transcription and mitochondrial function. SCF promotes thermogenesis and suppresses weight gain Kitl expression in BAT is altered in pathological conditions ( Fig. 1 ), and this led us to ask whether Kitl expression is also sensitive to physiological cues. Two alternative splice forms of Kitl exist in most tissues. The longer transcript contains a proteolytic cleavage site in exon 6 and is cleaved to generate a soluble isoform (sSCF), while the shorter transcript lacks exon 6 and stays membrane-bound (mSCF) [22] . We found that levels of both soluble and total Kitl transcripts in BAT increase after refeeding of overnight-fasted mice. The ratio of soluble to total Kitl also significantly increases ( Fig. 8a ). We also observed an increase in serum level of SCF in refed mice ( Fig. 8b ). Overnight exposure of mice to cold also increases the level and ratio of soluble Kitl in BAT ( Fig. 8c ). Although serum SCF remains the same in cold-challenged mice ( Fig. 8d ), local SCF level in BAT is significantly increased after cold exposure ( Fig. 8e ). In addition, we compared the Kitl expression in BAT of mice housed at either thermoneutrality (30 °C) or cold (6 °C) for 7 days, and found that there is a more substantial increase in the level and ratio of soluble Kitl , comparing cold to thermoneutrality ( Fig. 8f ). These data indicate that SCF potentially plays an important role in diet- and cold-induced thermogenesis. 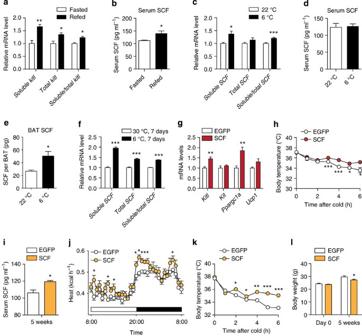Figure 8: SCF overexpression increases thermogenesis. (a) Soluble and totalKitlmRNA levels in BAT and (b) serum SCF levels from overnight-fasted and 3 h refed mice (n=4). (c) Soluble and totalKitlmRNA levels in BAT and (d) serum SCF levels from mice exposed to ambient temperature (22 °C) or cold (6 °C) for 24 h (n=4). (e) SCF level in BAT from cold-challenged mice (n=4). (f) Soluble and totalKitlmRNA levels in BAT from mice acclimated at thermoneutrality (30 °C) or cold (4 °C) for 7 days. (g,h) Lentiviruses expressing EGFP (n=6) or SCF (n=11) were injected into interscapular BAT of 8-week-old male C56BL/6 mice (1 × 106transforming units per site). Four weeks later, gene expression in BAT (g) and body temperature during cold exposure (h) were determined. (i–l) Lentiviruses expressing EGFP (n=4) or SCF (n=5) (1 × 106transforming unit per mouse) were administrated via the tail vein. Serum SCF level (i), energy expenditure (j), body temperature during cold exposure (k) and body weight (l) were determined 5 weeks later. Data are shown as mean±s.e.m. *P<0.05; **P<0.01; ***P<0.001 by two-tailed Student’st-test. Figure 8: SCF overexpression increases thermogenesis. ( a ) Soluble and total Kitl mRNA levels in BAT and ( b ) serum SCF levels from overnight-fasted and 3 h refed mice ( n =4). ( c ) Soluble and total Kitl mRNA levels in BAT and ( d ) serum SCF levels from mice exposed to ambient temperature (22 °C) or cold (6 °C) for 24 h ( n =4). ( e ) SCF level in BAT from cold-challenged mice ( n =4). ( f ) Soluble and total Kitl mRNA levels in BAT from mice acclimated at thermoneutrality (30 °C) or cold (4 °C) for 7 days. ( g , h ) Lentiviruses expressing EGFP ( n =6) or SCF ( n =11) were injected into interscapular BAT of 8-week-old male C56BL/6 mice (1 × 10 6 transforming units per site). Four weeks later, gene expression in BAT ( g ) and body temperature during cold exposure ( h ) were determined. ( i – l ) Lentiviruses expressing EGFP ( n =4) or SCF ( n =5) (1 × 10 6 transforming unit per mouse) were administrated via the tail vein. Serum SCF level ( i ), energy expenditure ( j ), body temperature during cold exposure ( k ) and body weight ( l ) were determined 5 weeks later. Data are shown as mean±s.e.m. * P <0.05; ** P <0.01; *** P <0.001 by two-tailed Student’s t -test. Full size image To test the function of SCF in vivo , we first overexpressed SCF in BAT by locally injecting lentiviruses encoding EGFP or SCF. The expression of inflammatory markers is similar between the two groups ( Supplementary Fig. 4a ). Compared with the EGFP control, SCF overexpression significantly increases Ppargc1a transcription, though the expression of Kit and Ucp1 is not affected ( Fig. 8g ). Moreover, SCF-overexpressed mice show higher body temperature during cold exposure, indicating increased thermogenesis in these mice ( Fig. 8h ). We also injected the lentiviruses though the tail vein to obtain systemic overexpression of SCF, and asked whether an increase in serum SCF is beneficial to mice ( Fig. 8i ). SCF viral overexpression increases the levels of Ppargc1a mRNA in both BAT and soleus muscle, without affecting the expression of inflammatory markers ( Supplementary Fig. 4b–d ). As expected, systemic administration of SCF increases energy expenditure in mice, without affecting food intake, RER or locomotor activity ( Fig. 8j and Supplementary Fig. 4e–g ). As a result, SCF-overexpressed mice are protected from cold-induced decrease in body temperature ( Fig. 8k ) and gain less weight over time ( Fig. 8l ). These data indicate that SCF is a potential therapeutic target for obesity. Mitochondria are not just the cell’s powerhouse for energy production, but are also responsible for heat production, initiation of apoptosis and regulation of cell signalling [1] , [29] . Mitochondrial dysfunction is associated with obesity, diabetes and ageing, though it is still unclear whether mitochondrial abnormalities are the cause or the consequence of these metabolic disorders [10] . Here, by analysing a mouse strain with a mutation in Kit gene, we demonstrate that SCF/Kit controls mitochondrial function and energy expenditure through the regulation of Ppargc1a transcription. The mutant mice develop obesity and glucose imbalance as a result of mitochondrial dysfunction and reduced energy expenditure. The defects in mitochondrial function in multiple tissues precede the onset of obesity, arguing that mitochondrial dysfunction can be a direct cause of metabolic diseases. SCF and Kit have been extensively demonstrated to regulate multiple cell lineages including melanocytes, germ cells, haematopoietic cells and mast cells. Loss-of-function mutations in either gene lead to deficiencies/defects in these cells [23] . Studies of the roles of SCF/Kit pathway in metabolism are emerging. Kit plays an important role in β-cell development, and Kit W−v mutant mice exhibit impaired glucose tolerance associated with decreased insulin secretion [30] . Kit also controls lipid metabolism in the liver, and mutations in Kit ( Kit Sco5 and Kit W/W−v ) induce juvenile steatosis in mice [31] . Here we demonstrate that Kit promotes PGC-1α expression and mitochondrial function, and Kit Wads and Kit Wps mutant mice are obese. On the other hand, mast cells have been shown to promote protease expression and microvessel growth in WAT, and mast cell-deficient Kit W−sh mice show reduced body weight and improved glucose homeostasis [32] . The variable and somehow contradictory phenotypes observed may be attributed to the nature of Kit mutations in these strains. For instance, Kit W mice carry a hypomorphic point mutation that affects splicing of Kit mRNA in various tissues [33] . The Kit W−sh allele is an inversion located proximal to the Kit gene that disrupts 5' regulatory sequences and also has been shown to affect the expression of neighbouring genes [34] . We also noticed that previous studies were conducted in mice that have different genetic backgrounds from the C57BL/6 mice that we used. Recently, a cocktail of haematopoietins including SCF was shown to promote the differentiation of human pluripotent stem cells into functioning brown adipocytes [24] . Our current study provides further evidence of the critical role of SCF/Kit signalling in BAT physiology. BAT and UCP1 are critical for adaptive thermogenesis [6] . However, we could not detect any decrease in Ucp1 mRNA in BAT or other tissues in Wps / Wps mice. We were then able to demonstrate decreased PGC-1α expression and mitochondrial function in thermogenic tissues including BAT, WAT and skeletal muscle. However, further experiments are necessary to determine the metabolic regulation by SCF/Kit signalling in individual tissues, and their relative contribution to energy expenditure. In line with our observations, PGC-1α knockout mice develop mitochondrial dysfunction, cold intolerance and obesity in the absence of change in UCP1 expression [16] . Increased mitochondrial oxidation in adipose tissue by Tfam knockout increases energy expenditure and protects mice against obesity and insulin resistance, also in a UCP1-independent manner [35] . We have shown that SCF/Kit signalling directly modulates Ppargc1a transcription through PI3K/Akt and MEK/Erk pathways. There are additional molecular links that may exist between SCF/Kit and PGC-1α. For example, PI3K/Akt regulates the expression of ERRα and mitochondrial function [36] . Activation of PI3K/Akt by PTEN deletion is associated with increased mitochondrial mass and respiration [36] . p38 MAPK and Ca 2+ signalling has been shown to drive activation of Ppargc1a transcription by exercise and cold [11] , and stimulation of SCF/Kit is known to activate p38 and Ca 2+ mobilization [22] . Therefore, it is possible that SCF/Kit signalling also modulates Ppargc1a transcription through p38-, Ca 2+ signalling-, or ERRα-dependent pathways. Expression of SCF/Kit is responsive to feeding/fasting cycles and cold exposure and is altered in obese mice and humans. We believe that released SCF will mediate diet- and cold-induced thermogenesis and promote heat production to combat the positive energy balance in obesity. This is confirmed by the finding that BAT-specific or systemic administration of SCF promotes thermogenesis and improves energy homeostasis in mice. Defining the mechanisms by which hormones and environmental cues dictate the expression of SCF/Kit in metabolic tissues will be an important avenue of future research. Bone morphogenetic protein 4 (BMP4) has been shown to upregulate Kit gene expression [37] , and BMP4 in WAT induces Ppargc1a expression, mitochondrial biogenesis and energy expenditure in WAT [38] . It would be interesting to determine whether BMP4 takes effect in adipose tissue through modulating Kit expression. With this knowledge, the SCF/Kit pathway can be considered as a potential therapeutic target for treating obesity and related metabolic diseases. Human samples Twelve subjects, all Han Chinese, were recruited at Drum Tower Hospital Affiliated to Medical School of Nanjing University. The study was approved by the ethics committee of the Medical School of Nanjing University, and informed consent was obtained from every participant. Animals Mice of C57BL/6J background were free to access water and either fed on a standard chow diet or 60% HFD (Research Diets). All procedures were conducted with the approval of the IACUC of Model Animal Research Center of Nanjing University. Body weights were recorded every week. For food intake test, mice were individually housed for at least 1 week for environmental habituation, and food consumption was weighed every morning for 7 consecutive days. For assessment of fat and lean mass, mice were examined with the PIXImus small animal dual-energy X-ray absorptiometry system (GE). Indirect calorimetry and metabolic assays Mice were housed individually in Comprehensive Lab Animal Monitoring System (Columbus Instruments). After 2 days to allow for adaptation, O 2 , CO 2 and activity were measured continuously for at least 3 days. Core body temperatures were measured rectally using a themo-coupler (Physitemp). Heat production was calculated and adjusted to body weight using ANCOVA analysis [39] . Serum was collected, and then analysed for leptin (Crystal Chem) and SCF (R&D) using ELISA Kits. For glucose tolerance tests, overnight-fasted mice were injected intraperitoneally with 2 g glucose per kg of body weight. For insulin tolerance tests, mice were fasted for 6 h and injected with 0.75 IU per kg human Insulin (Novo Nordisk). Blood samples were collected from tails and measured for glucose concentration with a glucometer (Arkray). Histology Adipose tissues were isolated and fixed in 4% paraformaldehyde and sectioned. Haematoxylin & eosin (H&E) staining was performed routinely. For TEM, tissues were quickly dissected and fixed in phosphate-buffered 2.5% glutaraldehyde, and the TEM was carried out at Nantong University using Jem-100s TEM (JEOL). Pre-brown adipocyte isolation and culture Four-week-old mice of different genotypes were killed, and their interscapular brown fat pads were minced and digested using Collagenase A (CLS004196, Worthington). The digested tissues were seeded in DMEM+10% FBS after being filtered through 100-μm filters. Twenty-four hours later, the adherent pre-brown adipocytes were immortalized by a lentivirus express SV40 largeT antigen (Genomeditech, Shanghai, China.). Immortalized pre-adipocytes were plated in DMEM containing 10% FBS, 20 nM insulin and 1 nM T4. After confluence, cells were stimulated with DMEM containing 10% FBS, 20 nM insulin, 1 nM T3, 0.5 mM isobutylmethylxanthine, 2 μg ml −1 dexamethasone and 0.125 mM indomethacin for 2 days, and then switched back to DMEM containing 10% FBS, 20 nM insulin and 1 nM T3 for 2–4 days until fat droplet appeared. 3T3-L1 cells were cultured in DMEM medium supplemented with 10% FBS, penicillin and streptomycin. Cells were overnight-fasted in DMEM + 0.5% BSA and pretreated with the following reagents: 0.8 ng ml −1 Rapamycin (mTOR inhibitor), 10 μM U0126 (MEK inhibitor), 50 nM Wortmannin (PI3K inhibitor) or 100 μM ZSTK474 (selective PI3K inhibitor) and then 100 ng ml −1 SCF for 12 h. Lentiviral injection The recombinant lentivirus for SCF-2A-EGFP, which expresses the first six exons of soluble mouse SCF in frame with 2A sequences and EGFP, was purchased from Genechem (Shanghai, China). C57BL6 mice (8-week-old male) were infected with lentiviruses (1 × 10 6 infection unit per mouse) by injection through tail vein or directly into the interscapular BAT. Real-time PCR RNA from tissues or cells was isolated using RNAiso (TaKaRa), and reverse transcription was carried out using first strand cDNA synthesis Kit (TaKaRa). Real-time PCR was analysed using EvaGreen dye (Biotium) in an ABI 7700 sequence detector (Applied Biosystems). Primer sequences are summarized in Supplementary Table 1 . Mitochondria isolation and oxygen respiration Tissue mitochondria were isolated using Sigma’s mitochondria isolation kit. The respiration rate of isolated mitochondria was measured using a Hansatech Clark-type oxygen electrode in the reaction medium (120 mM KCl, 20 mM sucrose, 3 mM HEPES, 2 mM KH2PO4, 2 mM MgCl2, 2 mM EGTA, pH 7.2) at 37 °C. For BAT mitochondria, oxygen consumption was determined in the presence of 10 μM rotenone, 10 mM succinate and 5 μM oligomycin. State III respiration rate of soleus mitochondria was determined in the presence of 10 μM rotenone, 10 mM succinate and 200 μM ADP. Western blotting and antibodies Tissue proteins were extracted using 1% Nonidet P-40, 50 mM Tris·HCl, 0.1 mM EDTA, 150 mM NaCl, 1 mM DTT, 0.4 mM PMSF, 0.1 mM Na 3 VO 4 and proteinase inhibitors. Protein concentrations were determined using BCA Protein Assay Kit (Pierce). Equal amounts of protein samples were subjected to western blot. The following antibodies were used: PGC1α (Abcam, ab54481, 1: 500 dilution), phospho-Erk1/2 (Y204) (Bioworld, BS4621, 1: 500 dilution), Erk1/2 (L352) (Bioworld, BS1112, 1: 500 dilution), phospho-Tyr (PY20) (Santa Cruz Biotechnology, sc-508, 1: 500 dilution), c-Myc (9E10) (Santa Cruz Biotechnology, sc-40, 1: 500 dilution), β-Actin (AC-15) (Sigma, A5441, 1: 10,000 dilution), α-Tubulin (B-5-1-2) (Sigma, T5168, 1: 10,000 dilution), phospho-Akt (Cell Signaling Technology, 9271, 1:1,000 dilution) and Akt (Cell Signaling Technology, 4691, 1:1,000 dilution). Full-size images of blots are shown in Supplementary Fig. 5 . Statistical analysis Data are presented as mean±s.e.m. The comparisons between two groups were carried out using two-tailed unpaired Student’s t -test. For multiple-group comparisons, one-way ANOVAs were used to test for no differences among the group means. Post hoc comparisons were adjusted using Bonferroni corrections. How to cite this article: Huang, Z. et al . The stem cell factor/Kit signalling pathway regulates mitochondrial function and energy expenditure. Nat. Commun. 5:4282 doi: 10.1038/ncomms5282 (2014).